MARQUIS: A multiplex method for absolute quantification of peptides and posttranslational modifications Absolute quantification of protein expression and posttranslational modifications by mass spectrometry has been challenging due to a variety of factors, including the potentially large dynamic range of phosphorylation response. To address these issues, we have developed MARQUIS—Multiplex Absolute Regressed Quantification with Internal Standards—a novel mass spectrometry-based approach using a combination of isobaric tags and heavy-labelled standard peptides, to construct internal standard curves for peptides derived from key nodes in signal transduction networks. We applied MARQUIS to quantify phosphorylation dynamics within the EGFR network at multiple time points following stimulation with several ligands, enabling a quantitative comparison of EGFR phosphorylation sites and demonstrating that receptor phosphorylation is qualitatively similar but quantitatively distinct for each EGFR ligand tested. MARQUIS was also applied to quantify the effect of EGFR kinase inhibition on glioblastoma patient-derived xenografts. MARQUIS is a versatile method, broadly applicable and extendable to multiple mass spectrometric platforms. Innovations over the past decade in methodology and instrumentation have greatly increased the capability of mass spectrometry (MS) to identify a significant fraction of the proteome, including thousands of posttranslational modifications (PTMs) [1] . Through the use of quantitative strategies, including label-free proteomics, metabolic-stable isotope labelling and chemical-stable isotope labelling, it is possible to analyse two or more biological samples and generate relative quantification data, detailing differences in protein expression or modification across different cellular conditions [2] , [3] . Multiplex labelling has effectively improved the throughput of the approach, enabling the comparison of multiple different biological samples in a single analysis, with quantification typically determined relative to a basal condition or pooled standard. Multiplexed relative quantification has been useful for elucidating temporal dynamics of phosphorylation signalling following growth factor stimulation, with changes in protein PTM levels in stimulated versus non-stimulated conditions highlighting pathways involved in signal processing and cellular response [4] . When combined with bioinformatic algorithms, such as clustering, relative quantification of PTM level has enabled researchers to predict the function of poorly characterized phosphorylation sites [5] . Through quantification of downstream biological response and statistical analysis, key sites have been identified as regulators of observed cellular behaviour, providing further functional and phenotypic association for novel phosphorylation sites [6] . Despite the ability to generate biological insight with a combination of relative quantification of phosphorylation dynamics and statistical modelling or bioinformatics, additional information is encoded in the absolute levels of site-specific phosphorylation. For instance, relative fold change of a signal carries limited information about the network’s basal state or response to stimuli, as a twofold change from a high basal state (for example, 30% to 60% activation) can lead to a very different biological response from a twofold change from a very low basal state (for example, 1% to 2% activation). Absolute quantification also enables comparison between multiple phosphorylation sites on a given protein under different conditions. As each phosphorylation site might recruit adaptor proteins associated with particular signalling pathways, absolute quantification of phosphorylation can provide critical data relating receptor stimulation and pathway activation. Absolute quantification of phosphorylation incorporation has historically been performed by using radiolabelled ATP and tryptic digestion followed by two-dimensional thin-layer chromatography; however, it is difficult to identify the specific phosphorylation sites corresponding to each peptide, the method is limited to single protein analysis and the phosphorylation reaction must occur in vitro (in cell lysates) or in cells whose membranes have been disrupted. In considering more high-throughput techniques, absolute quantification data is not typically available from standard MS, western blotting or reverse-phase protein array experiments, as the calibration curve is unique to each phosphorylated peptide due to different response profiles (for example, ionization potential or antibody-binding affinity). Therefore, multiple methods for estimating absolute quantification have been established. Among these, one of the most common MS-based methods is isotope dilution, or AQUA, in which a synthetic isotope-encoded peptide is added to the sample pre-analysis and quantification is based on the relative peak heights or area under the chromatographic elution curve for the endogenous and synthetic peptide standard [7] . Although this technique is fairly straightforward, it relies on single-point calibration and may provide erroneous estimates if the endogenous peptides span a large dynamic range across multiple conditions, or if the concentrations of these peptides fall outside of the linear response range of the instrument. Alternate methods for absolute quantification include the generation of standard curves through separate analyses of standard peptides at known concentration [7] . As the complex background of the biological context can significantly alter the signal intensity of the endogenous peptide due to competition for charge in the ionization process in MS, comparison with a standard curve generated in a neat background can lead to significant estimation errors. One solution would include different concentrations of a standard peptide into the sample so that the standard and endogenous peptides experience the same local sample context, but then one is faced with the issue of differentiating the standards from the endogenous peptides. Ideally, one would like to combine the multiplexed capabilities of chemical labelling with standard curves internal to the sample, thus allowing the accurate, absolute quantification of given peptides across multiple biological conditions within a single analysis. With these goals in mind, we have developed Multiplex Absolute Regressed Quantification of Internal Standards (MARQUIS), an MS-based technique to measure the absolute amount of modification on many posttranslational sites of interest simultaneously from multiple samples within a single analysis. The method uses multiple doses of internal standards to bracket a broad abundance range, allowing simultaneous analysis of treatment conditions expected to produce widely varied endogenous signal magnitudes. We applied MARQUIS to quantify the absolute amount of phosphorylation on several sites in the epidermal growth factor receptor (EGFR) network at different time points following stimulation of EGFR with different ligands. Absolute quantification of phosphorylation dynamics in this system highlights novel wiring within the network, insight that was not previously available from relative quantification data. MARQUIS enables the acquisition of accurate absolute quantification data, is applicable across multiple instrument platforms and is equally applicable to protein expression profiling and PTM quantification. Assessing the requirement for standard peptides To assess the need for internal standards, we selected several tyrosine phosphorylation sites in the EGFR signalling network, generated synthetic phosphorylated peptides encompassing these sites and added these peptides at defined concentrations to cell lysate of MCF10A cells. Quantification of the signal intensity for each peptide across multiple different analyses demonstrated a significant amount of run-to-run variation (three representative examples are presented in Fig. 1 ), probably associated with small flow-rate fluctuations combined with differences in temporal sampling across the chromatographic elution profile. To quantify this data across multiple concentrations of each peptide, we calculated the response ratio, the ratio between signal amplitude and peptide concentration, for 13 peptides in the EGFR signalling network ( Supplementary Fig. 1 ). As the data demonstrates, for a given concentration the response ratio can vary by two to three orders of magnitude. This variation is probably associated with differences in ionization potential of the peptides and their respective co-eluting species, due to competition for charge in electrospray ionization. Together, the broad range in peptide-specific response ratio and the technical replicate variation make it difficult to directly relate signal intensity and abundance, thereby highlighting the need for an improved method to generate accurate absolute quantification data. 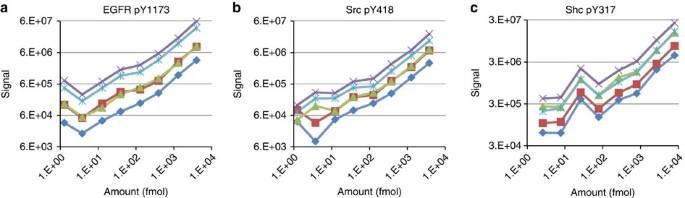Figure 1: Variability of signal intensity from technical replicates. The signal intensity versus amount of peptide is plotted for three representative peptides: EGFR pY1173 (a), Src pY418 (b) and Shc pY317 (c) across five technical replicate analyses. Figure 1: Variability of signal intensity from technical replicates. The signal intensity versus amount of peptide is plotted for three representative peptides: EGFR pY1173 ( a ), Src pY418 ( b ) and Shc pY317 ( c ) across five technical replicate analyses. Full size image The MARQUIS method for absolute quantification To quantify the absolute levels of endogenous peptides across a broad dynamic range, we have developed the MARQUIS method. Absolute quantification in MARQUIS is based on comparison of the endogenous peptides with paired heavy-isotope-labelled internal standards added at specific concentrations into multiple biological samples ( Fig. 2 ). Briefly, synthetic peptides containing a heavy-isotope-labelled amino acid were generated for each phosphorylated peptide of interest and stock concentrations were established by amino-acid analysis (AAA). A standard peptide cocktail was then added to cell lysates, one concentration per lysate. These lysates were purified and digested before stable isotope labelling (isotopic tags for relative and absolute quantification (iTRAQ)) and combination. The mix of endogenous and synthetic peptides was subjected to targeted tandem MS (MS/MS) for iTRAQ quantification and peptide sequence confirmation. Sequence-specific transitions were chosen based on previously observed fragmentation of the same peptides. Isobaric phospho-isoforms of the same peptide did not co-elute, enabling quantification of each isoform. Fragmentation of the iTRAQ-labelled synthetic, heavy-labelled phosphopeptide produced an internal standard curve, with each calibration point corresponding to the unique amount of synthetic peptide added to the corresponding biological sample. Similarly, fragmentation of the iTRAQ-labelled endogenous peptide also produced iTRAQ marker ions, with the intensity of each ion corresponding to the amount of endogenous peptide in each biological sample. Calibration of the iTRAQ marker ion intensities from the endogenous peptide against the standard curve provided absolute quantification for each biological condition. The internal standard curve establishes the linear dynamic range around the endogenous peptide concentration, providing an accurate intrinsic quality assessment of the peptide quantification. 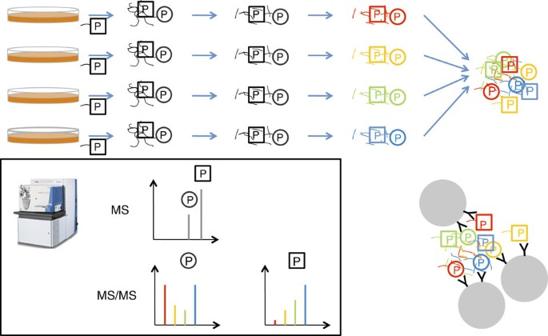Figure 2: MARQUIS method for absolute quantification. Synthetic isotope-labelled phosphorylated peptides (represented by the square box) are added during cell lysis. Following sample processing and digestion, all peptides, synthetic and endogenous (represented by the circle), are iTRAQ labelled. For this particular application of the method, tyrosine-phosphorylated peptides are enriched by peptide immunoprecipitation followed by immobilized metal affinity chromatography (IMAC), and analysed by LC–MS/MS. Heavy-labelled standards provide an internal calibration curve, enabling absolute quantification of endogenous peptides. Figure 2: MARQUIS method for absolute quantification. Synthetic isotope-labelled phosphorylated peptides (represented by the square box) are added during cell lysis. Following sample processing and digestion, all peptides, synthetic and endogenous (represented by the circle), are iTRAQ labelled. For this particular application of the method, tyrosine-phosphorylated peptides are enriched by peptide immunoprecipitation followed by immobilized metal affinity chromatography (IMAC), and analysed by LC–MS/MS. Heavy-labelled standards provide an internal calibration curve, enabling absolute quantification of endogenous peptides. Full size image As synthetic peptides are added early in the processing workflow, losses are identical for the endogenous and synthetic peptides, as both experience identical environments through all post-digestion stages of preparation. Moreover, as the endogenous and heavy-labelled peptides co-elute, the peptides experience identical chromatographic and ionization contexts, removing an additional potential source of quantification error. Performance of the method To assess the performance of the MARQUIS method, heavy-labelled synthetic phosphorylated peptides were generated for selected tyrosine phosphorylation sites in the EGFR signalling network. Synthetic peptides were added to EGF-stimulated MCF10A cell lysate, thereby providing a complex, biologically relevant background for testing the response profile, linear dynamic range and sensitivity of this method. MARQUIS was initially evaluated on a triple quadrupole instrument operating in multiple reaction monitoring (MRM) mode, with ten precursor-fragment ion transitions per peptide, including two sequence-specific and eight iTRAQ marker ion transitions ( Supplementary Figs 2 and 3 , and Supplementary Table 1 ). It is important to note that the number of phosphorylation sites able to be monitored with this approach is inherently limited by the number of transitions. With ten transitions per peptide and two peptides (synthetic and endogenous) per phosphorylation site, the total number of transitions increases rapidly as more sites in the network are monitored. Increasing the number of transitions translates to fewer measurements per peptide across the chromatographic elution profile, leading to sub-optimal quantitative data. To address this issue, we also evaluated MARQUIS on an Orbitrap-based instrument (QExactive) using targeted MS/MS, also known as parallel reaction monitoring (PRM). In this approach, a full-scan, high-resolution MS spectrum is acquired, followed by full-scan, high-resolution MS/MS spectra containing both iTRAQ marker ions and sequence-specific peptide fragmentation for each peptide ( Supplementary Fig. 4 ). As the endogenous and heavy-labelled peptides are both detected in the MS scan, quantitative comparison of the precursor ion intensities provides an estimate of the total amount of endogenous peptide present in the sample ( Supplementary Table 2 ). The relative iTRAQ marker ion intensities from the MS/MS spectrum for the endogenous peptide then apportion this total amount across the biological samples. iTRAQ marker ion intensities from the MS/MS of the standard peptide serve as an important control by providing a peptide-specific estimate of the accuracy and linear dynamic range. 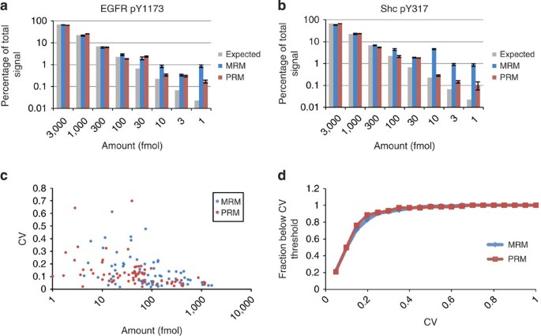Figure 3: Quality comparison of MARQUIS on the MRM versus PRM platform. Observed versus expected total iTRAQ signal contribution for MRM and PRM methods for two sites: EGFR pY1173 (a) and Shc pY317 (b). Data represents mean and s.d. across five technical replicates. (c) CV versus amount for MRM and PRM methods. (d) Fraction of measurements that meet CV thresholds for both techniques. For both the MRM and PRM methods, we selected 13 phosphorylation sites to assess the performance of MARQUIS quantification at different peptide concentrations (full data available in Supplementary Table 3 , representative temporal data for two peptides are plotted in Supplementary Fig. 5 ). Representative data extracted for two standard peptides using MRM and PRM is shown in Fig. 3 . At the high end of the curve, both methods perform identically. For EGFR pY1173 ( Fig. 3a ), the linear range for both MRM and PRM extends from 3,000 to 100 fmol; between 100 and 3 fmol, the response remains linear, but deviates from the theoretical response due to additional noise in the experimental measurement. For Shc pY317 ( Fig. 3b ), the PRM method performs well with a dynamic range of ~1,000-fold (3,000 to 3 fmol). The MRM method for this site did not perform as well, with suspected contamination on the iTRAQ-118 (10 fmol) channel boosting the recorded intensity significantly. This contamination does not appear to affect the iTRAQ-119 (3 fmol) or iTRAQ-121 (1 fmol) channels, as both show measurably lower values than iTRAQ-117 (30 fmol). Contamination may appear in the MRM method and not the PRM method due to the ability of the high-resolution PRM method to distinguish contaminant ions from iTRAQ marker ions, whereas the MRM measurement detects the number of ions passing a set bandwidth in the third quadrupole. It is worth noting that altering the dwell time per transition for MRM or the ion target value and maximum fill time for the PRM method can affect the sensitivity of the analysis and thereby improve the linear dynamic range, but increasing these values comes at the expense of cycle time. Figure 3: Quality comparison of MARQUIS on the MRM versus PRM platform. Observed versus expected total iTRAQ signal contribution for MRM and PRM methods for two sites: EGFR pY1173 ( a ) and Shc pY317 ( b ). Data represents mean and s.d. across five technical replicates. ( c ) CV versus amount for MRM and PRM methods. ( d ) Fraction of measurements that meet CV thresholds for both techniques. Full size image To evaluate the reproducibility of quantification using the MARQUIS method, we performed technical replicates of each experiment on the MRM and PRM platforms, and plotted the concentration versus coefficient of variation (CV) for each measurement in the data set ( Fig. 3c ). Although both methods provide high-quality data (for example, most measurements have CV <0.15) across the entire range, the most reproducible measurements are obtained above 100 fmol, with CV values <0.1. At the low end of the concentration range, some peptides display CV >0.5. For MRM, the early time points of ERK1 and ERK2 signals exhibited the highest CV, probably due to the combination of low endogenous signal coupled to the higher standard doses included in the corresponding channels. Inclusion of a second heavy-labelled amino acid residue would increase the spacing between the endogenous and standard peptides, and thereby decrease the potential issue of isolation window contamination. The highest CVs for the PRM technique were those of the dual phosphorylated EGFR peptide pY1045/pY1068. This peptide has a lower response ratio ( Supplementary Fig. 1 ) and elutes very late in the chromatographic programme, making it more susceptible to contamination from background chemical noise. Overall, both techniques were comparable in terms of the fraction of measurements that met CV thresholds ( Fig. 3d ) at a CV of 0.20. Isolation width effects In the MARQUIS method, both the endogenous and the heavy-labelled synthetic peptides are iTRAQ labelled, allowing for direct comparison of iTRAQ marker ion intensities resulting from fragmentation of the corresponding peptides. This approach has the potential for error associated with contamination of the isolation window from other endogenous or synthetic peptides, or potentially from co-isolation of the endogenous and heavy-labelled peptides. As the charge state of the peptide increases, the separation, in m/z , between the endogenous and heavy-labelled synthetic peptide decreases, thereby increasing the likelihood of co-isolation. To assess the effect of the isolation width on MARQUIS quantification accuracy for the MRM platform, we narrowed the isolation width on the first quadrupole from 0.7 m/z to 0.1 m/z . Narrowing the MS1 isolation window can decrease the level of contamination in the ions selected for fragmentation, but also significantly decreases the transmission efficiency. To determine whether this trade-off was beneficial, we compared the measured signal intensities from all peptides from analyses run with both isolation widths ( Supplementary Fig. 6 ). Minimal effects of altered isolation width were seen for the highest peptide levels, whereas only the 0.1 m/z isolation window was able to clearly distinguish the median of the 1 fmol standard from the median of the 10 fmol standard. At the lowest peptide levels, the narrower isolation width was better able to isolate precursor ions, ultimately providing a larger dynamic range for calibration. However, for peptides with poor response ratios, the losses associated with the narrower isolation width ultimately limit the sensitivity and therefore the dynamic range. Tyrosine phosphorylation quantification in EGFR signalling Previous studies have described the temporal dynamics of individual tyrosine phosphorylation sites following EGFR activation [8] . Although these studies have highlighted many novel phosphorylation sites in the network and have led to hypotheses regarding the function of selected sites, they have been inherently limited by quantification relative to a selected time point. As such, it has been difficult to quantify differences in phosphorylation levels across different sites on the receptor, or to determine whether different ligands led to different phosphorylation stoichiometries. To address this deficiency and gain insight into the temporal phosphorylation profiles of multiple sites in the network, we used MARQUIS to quantify absolute levels of tyrosine phosphorylation on EGFR and proximal adaptor proteins, at multiple time points following EGF stimulation. Although EGFR pY1173 is often cited as a dominant autophosphorylation site for the receptor [9] and is often used as a measure of EGFR activation for immunoblotting studies [10] , [11] , MARQUIS data unequivocally demonstrates that phosphorylation of 1148 occurs ~4- to 5-fold greater than pY1173, pY1068 or pY1045, all of which occur at similar levels ( Fig. 4a ), a comparison that would be missed by typical MS-based relative quantification [6] or immunoblotting techniques. Further downstream in the network, it is also possible to detect higher levels of phosphorylation on Erk2 pY187 as compared with Erk1 pY204 ( Fig. 4b ), an observation that aligns with higher ERK2 expression in other systems [12] . 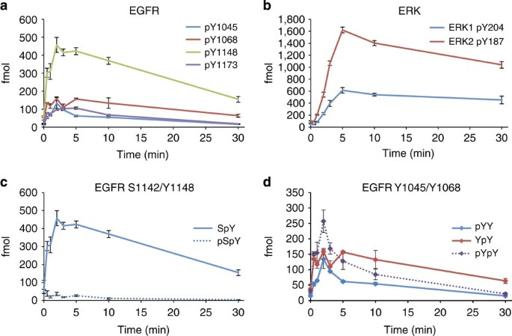Figure 4: Stoichiometric comparison of site-specific phosphorylation. Data for a collection of EGFR and network phosphorylation sites were gathered using MARQIS with MRM on a triple quadrupole instrument. (a) EGFR. (b) ERK1/2. (c) EGFR pY1148, pS1142/pY1148. (d) EGFR pY1045, pY1068 and pY1045/pY1068. Data represent mean and s.d. across three biological replicates. Figure 4: Stoichiometric comparison of site-specific phosphorylation. Data for a collection of EGFR and network phosphorylation sites were gathered using MARQIS with MRM on a triple quadrupole instrument. ( a ) EGFR. ( b ) ERK1/2. ( c ) EGFR pY1148, pS1142/pY1148. ( d ) EGFR pY1045, pY1068 and pY1045/pY1068. Data represent mean and s.d. across three biological replicates. Full size image Absolute quantification enables the tracking of individual phosphorylation sites, even when multiple sites are contained within the same tryptic peptide. For instance, the peptide containing Y1148 also contains S1142, a serine residue that has previously been found to be phosphorylated in these cells [13] . To identify whether pS1142 co-occurs with pY1148 on the same EGFR protein, we used MARQUIS for absolute quantification of the singly phosphorylated pY1148 peptide and the doubly phosphorylated pS1142/pY1148 peptide. By quantifying the singly and doubly phosphorylated isoforms of the peptide, we could more accurately account for the total amount of phosphorylation on Y1148 ( Fig. 4c ). This analysis led to the intriguing finding that pS1142/pY1148 is present in unstimulated cells at approximately the same level as the singly phosphorylated pY1148, but on stimulation gradually decreases over time. In comparison, the singly phosphorylated pY1148 increases strongly following EGF stimulation. With absolute quantification, it is clear that the increase in phosphorylation of the singly phosphorylated pY1148 is much greater than the decrease in the doubly phosphorylated pS1142/pY1148 peptide. Therefore, the increase in singly phosphorylated pY1148 is probably due to phosphorylation of EGFR in the absence of pS1142 rather than de-phosphorylation of the pS1142/pY1148 species. It remains to be determined whether pS1142 inhibits phosphorylation of Y1148, but our data would be consistent with this hypothesis. Additional insights into phosphorylation dynamics are available when multiple tyrosine phosphorylation events occur on a given tryptic peptide. For instance, Y1045 and Y1068 fall within the same tryptic fragment, and therefore yield four possible phosphorylation isoforms for the peptide (Y1045/Y1068, pY1045/Y1068, Y1045/pY1068 and pY1045/pY1068), three of which were monitored by MARQUIS-based absolute quantification ( Fig. 4d ). Although all three isoforms are present at similar, low levels in unstimulated MCF10A cells, following stimulation Y1045/pY1068 and doubly phosphorylated pY1045/pY1068 both rise rapidly in the first minute. The pY1045/Y1068 peptide increases gradually in the first minute, potentially indicating that this site is being converted to the pY1045/pY1068 form through rapid phosphorylation of Y1068. Interestingly, over the next several time points the singly phosphorylated Y1045/pY1068 isoform begins to decrease, while the pY1045/Y1068 and pY1045/pY1068 isoforms both increase strongly, indicating phosphorylation of Y1045 that is converting Y1045/pY1068 into the doubly phosphorylated form, which is the most abundant of the three isoforms in this early time period. Finally, by 5 min all three of the phospho-isoforms begin to decrease at similar rates, potentially indicating the activity of a common phosphatase. The quantitative interplay between these isoforms has not been previously documented due to a lack of absolute quantification of phosphorylation level on each of these sites under different stimulation conditions. MARQUIS-based absolute quantification was also used to quantify EGFR phosphorylation dynamics in response to different EGFR ligands. It has previously been documented that stimulation with EGF, transforming growth factor-α, or amphgiregulin leads to different downstream biological effects [14] , [15] , [16] , potentially due to qualitatively or quantitatively different signalling networks. To uncover the mechanism by which these different ligands activate different phenotypes, we quantified the temporal dynamics of phosphorylation levels on multiple sites on the receptor and several downstream adaptor or effector proteins in response to different concentrations of each ligand ( Supplementary Table 4 ). As can be seen in Fig. 5a–c , each ligand stimulates a rapid increase in receptor phosphorylation, albeit to different levels, with the Y1148 site consistently phosphorylated to a greater extent compared with the other three phosphorylation sites on the carboxy-terminal tail of the receptor. Given that each ligand has different binding affinities, the difference in the level of phosphorylation on the receptor may not be surprising. Intriguingly, despite the quantitative difference in the level of phosphorylation due to each ligand ( Fig. 5d ), the pattern of phosphorylation on the receptor is effectively invariant with regard to ligand identity, with pY1148>pY1068>pY1173>pY1045; this similarity in receptor pattern can best be visualized by normalizing all sites for a given ligand to the median amount of phosphorylation on the receptor ( Fig. 5e ). The consistent pattern of receptor phosphorylation at this ligand dose raises the intriguing possibility that biological response to different EGFR ligands may be encoded in the absolute level of phosphorylation on each site rather than through the phosphorylation of different sites on the receptor (for example, quantitative versus qualitative control of receptor tyrosine kinase (RTK) phosphorylation signalling networks). Interestingly, quantitative control at the receptor level results in altered phosphorylation patterns even on proximal adaptor proteins such as Gab1 ( Supplementary Table 4 ); the mechanism underlying these pattern changes is currently unknown, but it is likely to be that changes in the amount of phosphorylation at the receptor may affect recruitment of other enzymes (kinases/phosphatases) or steric competition for binding to the receptor, thus leading to different protein complex assembly. 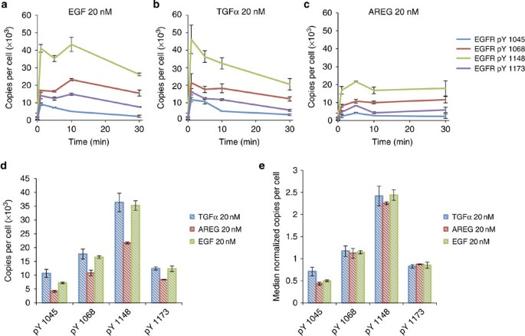Figure 5: Ligand comparison. MRM-based absolute quantification for EGFR phosphorylation sites treated with EGF (a), transforming growth factor-α (TGFα) (b) and amphgiregulin (AREG) (c). Comparison of site-specific phosphorylation between ligands following 5 min of ligand stimulation for two biological replicates; raw (d) and normalized (e). Data represent mean and range across two biological replicates. Figure 5: Ligand comparison. MRM-based absolute quantification for EGFR phosphorylation sites treated with EGF ( a ), transforming growth factor-α (TGFα) ( b ) and amphgiregulin (AREG) ( c ). Comparison of site-specific phosphorylation between ligands following 5 min of ligand stimulation for two biological replicates; raw ( d ) and normalized ( e ). Data represent mean and range across two biological replicates. Full size image Quantification of EGFR signalling in glioblastoma xenografts To assess the applicability of the MARQUIS method to the complex biological background represented by tissue samples, we chose a set of patient-derived xenografts (PDX) that vary in their EGFR expression and mutation profiles: GBM12 expresses a point mutation extracellular domain of EGFR; GBM6 and GBM39 express the constitutively active truncation mutant EGFR vIII; and GBM15 is EGFR wild-type amplified. Before searching for the endogenous signals, we confirmed that we could still build a large-dynamic-range standard curve in the more complex tumour background ( Supplementary Figs 7 and 8 ). In the worst cases, we were still able to cover at least two orders of magnitude, convincing us that we could adequately measure endogenous levels. With MARQUIS in PRM mode, we compared the absolute levels of phosphorylation for each EGFR phosphorylation site both within each PDX tumour model and across the various tumour models ( Fig. 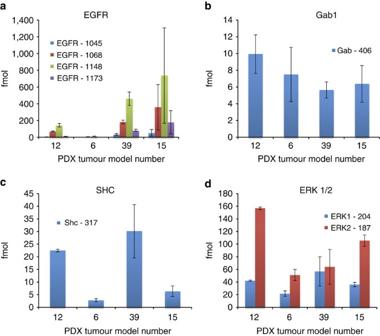Figure 6: Quantification of phosphorylation across four glioblastoma PDX tumour types. Absolute amounts of phosphorylation were quantified for each PDX mouse model of glioblastoma. Each tumour model was analysed in biological duplicate. EGFR (a). Gab1 (b). Shc (c). Erk1/2 (d). Data represent mean and range across two biological replicates. 6a and Supplementary Table 6 , (validated spectra for each quantification scan are included in Supplementary Fig. 9a–d )). For these PDX tumours, GBM6 (EGFRvIII) had the lowest level of EGFR phosphorylation, consistent with previous literature describing EGFRvIII as a weakly constitutively active kinase. Interestingly, GBM39 also expresses EGFRvIII, but is much more highly phosphorylated on the receptor. By comparison, GBM12 (EGFR point mutant) demonstrated an intermediate level of receptor phosphorylation and GBM15, the wild-type EGFR-amplified PDX tumour, had the highest level of phosphorylation. Large variation was observed in the different GBM15 tumour samples, potentially due to biological fluctuations between replicate tumours. Intriguingly, the pattern of EGFR phosphorylation was invariant when comparing the wild-type EGFR (GBM15) with the point mutant (GBM12) or the EGFRvIII mutation (GBM6 and GBM39), providing a separate example of quantitative versus qualitative regulation of receptor phosphorylation. For proximal adaptor proteins, little significant difference was observed in Gab1 Y406 phosphorylation ( Fig. 6b ), but Shc pY317 levels ( Fig. 6c ) were elevated for GBM12 and GBM 39 relative to GBM15 and GBM6, respectively. Downstream of SHC and GAB1, ERK2 was most highly phosphorylated in GBM12 and GBM15, while ERK1 phosphorylation levels were similar across all four GBM PDX tumours ( Fig. 6d ). It is worth noting that this data is in general agreement with our previous analysis of the signalling networks in these GBM PDX tumour lines [17] , except that MARQUIS provides absolute levels of quantification for the specific phosphorylation sites in each sample. Figure 6: Quantification of phosphorylation across four glioblastoma PDX tumour types. Absolute amounts of phosphorylation were quantified for each PDX mouse model of glioblastoma. Each tumour model was analysed in biological duplicate. EGFR ( a ). Gab1 ( b ). Shc ( c ). Erk1/2 ( d ). Data represent mean and range across two biological replicates. Full size image As an additional application, MARQUIS enables the absolute quantification of the effects of therapeutic treatment on tumour samples. In many cases, it is not known whether resistance arises due to failure to inhibit the target or due to compensatory signalling mechanisms. To quantify the effect of EGFR tyrosine kinase inhibitor treatment in vivo , GBM12 was treated with a panel of kinase inhibitors (erlotinib, dacomitinib, or NT-113), to compare the efficacy of a classic type 1 inhibitor (erlotinib) with the latest generation of covalent HER family inhibitors (dacomitinib and NT-113). Following tumour homogenization, the MARQUIS workflow was employed in PRM mode with the same heavy-labelled standard peptides and full-scan data collection liquid chromatography (LC)–MS (validated spectra for each quantification scan are included in Supplementary Fig. 8 ). The results of these analyses are presented in Fig. 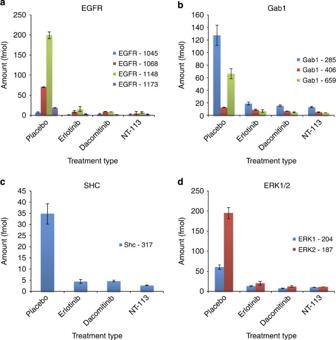Figure 7: Quantification of phosphorylation in a glioblastoma PDX treated with a panel of EGFR kinase inhibitors. Absolute amounts of phosphorylation were quantified in the GBM12 PDX tumours treated with placebo or one of three EGFR kinase inhibitors: erlotinib (100 mg kg−1), dacomitinib (10 mg kg−1) or NT-113 (15 mg kg−1). Each treatment condition was analysed in biological duplicate. EGFR (a). Gab1 (b). Shc (c). Erk1/2 (d). Data represent mean and range across two biological replicates. 7 and data are in Supplementary Table 7 . EGFR phosphorylation ( Fig. 7a ) in the placebo-treated tumours continues to resemble the patterns observed in the MCF10A cells treated with EGF. Following treatment with each of the inhibitors, EGFR phosphorylation on each site decreased significantly, by >90% on pY1068, pY1148 and pY1173, indicating effective inhibition of the target for each kinase inhibitor. Phosphorylation on the proximal adaptor proteins Gab1 pY285, Gab1 pY659 ( Fig. 7b ) and Shc pY317 ( Fig. 7c ) also decreased in response to each of the inhibitors, which corresponded to a decrease in Erk1 and Erk2 phosphorylation ( Fig. 7d ). None of the inhibitors had a significant impact on Src Y418 phosphorylation, but NT-113 decreased Shp2 phosphorylation on Y62 to a greater extent (~44% decrease) compared with dacominitib (~22%) and erlotinib (~10%). Figure 7: Quantification of phosphorylation in a glioblastoma PDX treated with a panel of EGFR kinase inhibitors. Absolute amounts of phosphorylation were quantified in the GBM12 PDX tumours treated with placebo or one of three EGFR kinase inhibitors: erlotinib (100 mg kg −1 ), dacomitinib (10 mg kg −1 ) or NT-113 (15 mg kg −1 ). Each treatment condition was analysed in biological duplicate. EGFR ( a ). Gab1 ( b ). Shc ( c ). Erk1/2 ( d ). Data represent mean and range across two biological replicates. Full size image MARQUIS is a novel multi-point internal standard calibration method that enables absolute quantification of site-specific PTM levels or protein expression. The method provides accurate quantification over a broad range of concentrations, allowing simultaneous analysis of stimulation conditions that lead to large changes in expression or modification levels. With MARQUIS, absolute quantification data can be collected for many PTM sites of interest in the network in a single analysis, using either MRM- or PRM-based targeted MS. This data can then be used for intra- and intersample site-specific comparisons. It is well known that isobaric labelling strategies such as iTRAQ or tandem mass tags (TMT) suffer from ratio compression in complex mixture analysis due to the inclusion of contaminating peptides during the isolation of the precursor peptide for fragmentation. Importantly, the MARQUIS method is novel in the inclusion of a standard curve within the biological sample, enabling the estimation of ratio compression at the same elution time as the endogenous peptides, and at a proximal mass-to-charge ratio. Thus, the MARQUIS method not only correctly estimates iTRAQ ratio compression but also enables compensation for that compression, a feature that is inherently lacking in most other absolute or relative quantification methods. It is also worth noting that the MARQUIS method enables accurate absolute quantification even for complex sample processing protocols before MS analysis. As synthetic phosphorylated peptides whose sequence matches exactly to the endogenous peptide are added during the cell lysis procedure, the MARQUIS method accounts for losses throughout post-digestion sample processing, including potentially inefficient immunoprecipitation of selected peptides or sub-optimal enrichment of phosphophorylated peptides. MARQUIS was designed for MRM-based analysis on a triple quadrupole, but the method is equally applicable to targeted full-scan targeted MS/MS (PRM). Overall, the two methods performed very well in terms of technical reproducibility with a CV threshold of 0.15 able to capture the majority of measurements with both techniques. Both instrument platforms offer selective advantages. For instance, the PRM method offers the ability to determine contamination by way of the complete MS/MS data at high resolution that is not available in an MRM experiment. On the other hand, when using MRM, the precursor (Q1) isolation window can be tightened to a greater extent compared with the PRM method, thereby improving signal-to-noise ratio by reducing contributions from spurious co-eluting ions. Although a Q1 isolation width of 0.7 m/z was typically used for the data acquired in this study, sufficient signal for quantification can be attained for many peptides by using a window as small as 0.1 m/z . Such a narrow window would be deleterious to the PRM method as the drop in ion flux may eliminate signal for most low- and medium-intensity fragments. The MRM approach is inherently more flexible, as the fragmentation energy and time spent per MRM transition can be altered for selected transitions to improve the sensitivity. However, increasing the dwell time is only feasible for a small number of transitions; otherwise, the increase in cycle time becomes too great. Recent structural insights into the cooperativity of ligand binding and EGFR dimerization suggest that differential ligand affinities for the extracellular portion of the receptor influence the occupancy and the receptor conformation, and potentially signalling and trafficking [18] . A previous MS-based study of receptor phosphorylation observed site-specific quantitative differences in receptor phosphorylation in response to varied doses of transforming growth factor-α and EGF; stoichiometry was estimated by measuring the ratio of signal intensities between phosphorylated and non-phosphorylated versions of tyrosine containing tryptic fragments [19] . Such comparisons are limited due to the differential ionization potential between these species. Here we have shown large differences not only between various ligand stimulation conditions for a single site, but also between different EGFR sites not present on the same tryptic peptide. The MARQUIS method enables quantification of EGFR phosphorylation stoichiometry, information necessary to decipher how extracellular ligand concentration information is transmitted across the cellular membrane. Unique sets of SH2- and PTB-containing proteins bind to each receptor phosphorylation site [20] , [21] , suggesting the ability to activate distinct pathways by phosphorylating different sites. Alternately, differential pathway activation could be controlled by altering the level of phosphorylation. Although this option might suggest that downstream pathways will be linearly proportional to receptor phosphorylation levels, different pathways feature amplification gains, and thus one pathway might be saturated by a relatively small signal on the receptor, as has been detected for the extracellular-signal-regulated kinase–mitogen-activated protein kinase (MAPK) pathway, while other pathways may be more analog in nature. Here, through absolute quantification of specific phosphorylation sites on the receptor, we determined that the EGFR phosphorylation response to stimulation with a relatively high concentration of different EGFR ligands is quantitatively regulated. Although phosphorylation levels are ligand specific, the ratio between different receptor sites is constant across different EGFR ligands. Thus, different biological responses may be regulated by the analog versus digital nature of the different downstream pathways, in a manner similar to the interleukin receptor system we have recently investigated [22] . Additional studies are needed to confirm the effects of quantitative regulation of receptor phosphorylation on downstream pathways, as well as to determine the cellular conditions that might lead to altered phosphorylation patterns on the receptor: is this a mechanism by which the cell differentiates normal versus pathological signalling? Finally, we have demonstrated the applicability of the MARQUIS method to generate absolute phosphorylation quantification data in tumour tissues. As MARQUIS provides absolute quantification in a multiplexed analysis, it enables quantification across different MS analyses, now providing the potential to generate absolute quantification of hundreds of tumour samples in a relatively small number of MS analyses. Furthermore, we have used MARQUIS to quantify the effects of therapeutic inhibition on these same tumour tissues. These data demonstrate the ability of MARQUIS to not only quantify the effect of different tyrosine kinase inhibitors (TKIs) on target phosphorylation levels, but also to quantify the effect of the inhibitor on proximal adaptor proteins, downstream effectors and off-target kinases. Absolute quantification of protein expression and PTM levels will be required to provide insight into regulation of many biological systems. The MARQUIS method enables facile acquisition of absolute quantification data across multiple biological conditions simultaneously, with large dynamic range, and with internal standard curves to improve the accuracy of the measurements. This method is broadly applicable to multiple MS platforms and to different biological systems. Sample preparation MCF10A cells (originally provided by the Brugge lab at Harvard Medical School) were serum starved 24 h before stimulation with 20 nM EGF (Peprotech) for 0.5, 1, 2, 3, 5, 10 or 30 min. Media was aspirated and cells were lysed with 2 ml of cold 8 M urea with 1 mM activated sodium orthovanadate. Lysate was frozen at −80 °C until further processing. Protein yield was quantified by BCA assay (Pierce) to ensure equal loading. Standard peptides were added to samples as in Supplementary Table 1 . Samples were reduced with 40 μl 10 mM dithothreitol in ammonium acetate pH 8.9 for 1 h at 56 °C. Samples were alkylated with 55 mM iodoacetamide in ammonium acetate pH 8.9 for 1 h at room temperature. 100 mM ammonium acetate and 40 μg of sequencing grade trypsin was added before 16 h incubation at room temperature. Lysates were acidified with 1 ml glacial acetic acid and protein was purified with Waters Sep-Pak columns. Samples were lyophilized and subsequently labelled with iTRAQ 8plex (AbSciex) as per the manufacturer’s directions. Standard peptide preparation and quality assurance Standard peptides were synthesized at the Koch Institute Biopolymers facility and amino acid analysis was performed to measure concentration by AAA Service Laboratories (Damascus, OR). Synthetic peptides were analyzsed by LC–MS/MS to confirm sequence and purity. Multiple reaction monitoring Immunoprecipitation . Seventy microlitres of protein G agarose beads (Calbiochem IP08) were rinsed in 400 μl Immunoprecipitation (IP) Buffer (100 mM tris, 0.3% NP-40, pH 7.4) before an 8 h incubation with a cocktail of three phosphotyrosine-specific antibodies (12 μg 4G10 (Millipore),12 μg PT66 (Sigma) and 12 μgPY100 (CST)) in 200 ml IP Buffer. Antibody cocktail was removed and beads were rinsed with 400 μl of IP Buffer. Labelled samples were resuspended in 150 μl iTRAQ IP Buffer (100 mM Tris, 1% NP-40, pH 7.4)+300 μl milliQ water and pH was adjusted to 7.4 (with 0.5 M Tris HCl, pH 8.5) before addition to prepared beads and 16 h incubation. Supernatant was removed and beads were rinsed three times with 400 μl Rinse Buffer (100 mM Tris HCl, pH 7.4). Peptides were eluted in 70 μl of Elution Buffer (100 mM glycine, pH 2) for 30 min at room temperature. Immobilized metal affinity chromatography purification . A fused silica capillary column (200 μm ID × 10 cm length) was packed with POROS 20MC beads (Applied Biosystems, catalogue number 1-5429-06). Column was rinsed with 100 mM EDTA, pH 8.9, in ultrapure water to remove residual iron and then rinsed with ultrapure water to remove EDTA before fresh iron was deposited by rinsing with 100 mM FeCl 3 in ultrapure water. Excess iron was removed with 0.1% acetic acid before loading the IP elution. The column was washed with 25% MeCN, 1% HOAc, 100 mM NaCl in ultrapure water to remove nonspecifically bound peptides and then rinsed with 0.1% HOAc. Peptides were eluted with 250 mM NaH 2 PO 4 in ultrapure water and collected on a pre-column (100 μm ID × 10 cm packed with 10 μm C18 beads (YMC gel, ODS-A, 12 nm, S-10 μm, AA12S11)). This pre-column was rinsed with 0.2 M acetic acid before LC–MS analysis. Liquid chromatography–mass spectrometry . The pre-column was connected in-line with an analytical column (50 μm ID × 10 cm packed with 5 μm beads (YMC gel, ODS-AQ, 12 nm, S-5 μm, AQ12S05)) with integrated electrospray emitter tip [23] . A 140-min gradient from aqueous (0.2 M acetic acid) and organic phase (0.2 M HOAc, 70% MeCN) was used to separate peptides with a flow rate of 200 nl min −1 and a flow split >99% and a spray voltage of 1,800 V. Isolation widths of 0.7 were used for both Q1 and Q3, and collected for 0.05 s. A width of 0.01 m/z was collected around each transition for quantification. Collision energies were determined per sequence with Thermo Pinpoint software. Absolute quantification . Analyses were performed on a Thermo TSQ Quantum in MRM mode. Endogenous and heavy-labelled versions of each peptide of interest were tracked throughout the experiment with two sequence-specific transitions (precursor/prominent b or y ion) and eight iTRAQ transitions (precursor/label peak). Elution time was determined based on co-elution of iTRAQ transitions with sequence-specific transitions for both standard and endogenous peptides of the MARQIS pair. Area under the curve (AUC) was collected for each transition. Data were corrected by iTRAQ isotope purity and synthetic peptide-loading control. A calibration curve was created for each peptide to relate the AUC of the iTRAQ transition to the amount of standard included. MATLAB function lscov was used with the intensity of the signal also serving to appropriately scale the variance. This calibration curve was then used to calculate the amount of peptide present in each of the endogenous conditions based on the corresponding iTRAQ transition AUC. Parallel reaction monitoring Immunoprecipitation . Twenty microlitres of protein G agarose beads (Calbiochem, IP04-1.5 ml) were pre-incubated with 20 μl of PT66 and 20 μl of pY100, before adding sample (reconstituted in 70 μl HEPES buffer adjusted with 5 M NaOH). After overnight incubation, beads were rinsed and peptides were eluted with 20 μl of 0.1% TFA, 10% MeCN, 250 ng μl −1 HeLa Digest (phospho depleted). NTA enrichment . Elution incubated with Fe(III)-NTA magnetic beads for 15 min, rinsed and eluted with 10 μl of NH 4 OH (1:30), 5 mM EDTA, 5% MeCN, 1 ng μl −1 HeLa digest. Elution was transferred to an autosampler vial and pH was adjusted with 5 μl of 10% TFA. Liquid chromatography–mass spectrometry . LC–MS was performed using a 25-cm, 75-μm ID, EASY-Spray column (ThermoFisher Scientific, ES802) with a 120-min gradient and a flow rate of 300 μl min −1 and a spray voltage of 1,800 V. Targeted MS2 scans were collected with a maximum ion injection time of 2 s and an AGC target of 3e6 with an MS1 isolation width of 1 m/z , and fragmented with a collision energy of 35.0. Absolute quantification (PTM method) . Analyses were performed on a Thermo Q-Exactive. Endogenous and heavy-labelled versions of each peptide were targeted for MS2 analysis during their expected elution times. In the MS1 scan, the total amount of endogenous peptide was calculated based on the fraction of MS1 integrated intensity when compared with the standard peptide. This amount was then apportioned across the contributing samples based on relative iTRAQ intensity. A single-point measurement where the MS2 scan used to determine the iTRAQ intensity ratios was chosen based on maximal MS1 intensity, to assure maximal signal-to-noise ratio. Tumour sample analysis All studies were reviewed and approved by the Mayo Institutional Animal Care and Use Committee. Subcutaneous xenografts for GBM 6, 12, 15 and 39 were established by injecting the flank of athymic nude mice with 1 × 10 6 cells suspended in Matrigel/PBS. Tumours were harvested and flash frozen in liquid nitrogen once they reached >1,500 mm 3 in size. For the GBM 12 pharmacodynamic study, 8 mice had flank tumours implanted and randomized into 4 treatment arms once the tumour reached at least 200 mm 3 in size: (1) placebo, (2) erlotinib 100 mg kg, (3) dacomitinib 10 mg kg, (4) NT-113 15 mg kg. A single dose was given to each mouse and the tumour was harvested at 6 h post treatment and flash frozen in liquid nitrogen. Five hundred micrograms of protein (as determined by BCA assay) from each tumour sample was processed as per the PRM LC–MS protocol following IP and immobilized metal affinity chromatography enrichment as previously described. Analyses were performed on a Thermo QExactive instrument fed by a Thermo Easy nLC1000 UPLC precolumn (Thermo 164705) and a self-pack PicoFrit analytical column (New Objective PF360-50-10-N-5) packed with 50 cm of 3 μm beads (ODS-AQ 12 nm, S-3 μm from YMC America AQ12S03). Samples were analysed on a 60-min gradient with a 200 nl min −1 flow rate; aqueous phase: 0.1% formic acid in HPLC-grade water; organic phase: 0.1% formic acid, 80% acetonitrile in HPLC-grade water. A spray voltage of 2,000 V was used. To ensure that the standard peptides did not contaminate the endogenous iTRAQ signals, each sample was run twice. Quantitative iTRAQ data for the endogenous peptides was collected from Sample A, as Sample A did not contain standard peptides that may potentially contaminate endogenous iTRAQ signal. MS/MS scans of endogenous peptides were collected with a 250-ms fill time, an AGC target value of 5e5 and an isolation window of 2 m/z . Quantitative iTRAQ data for the synthetic heavy-labelled standard peptides, as well as the ratio between standard and endogenous precursor peaks were collected from Sample B. MS/MS scans were optimized to collect the largest dynamic range possible by maximizing the fill time (3 s) and the AGC target (5e6). How to cite this article: Curran, T. G. et al . MARQUIS: A multiplex method for absolute quantification of peptides and posttranslational modifications. Nat. Commun. 6:5924 doi: 10.1038/ncomms6924 (2015).